Amino acid coevolution reveals three-dimensional structure and functional domains of insect odorant receptors Insect odorant receptors (ORs) comprise an enormous protein family that translates environmental chemical signals into neuronal electrical activity. These heptahelical receptors are proposed to function as ligand-gated ion channels and/or to act metabotropically as G protein-coupled receptors (GPCRs). Resolving their signalling mechanism has been hampered by the lack of tertiary structural information and primary sequence similarity to other proteins. We use amino acid evolutionary covariation across these ORs to define restraints on structural proximity of residue pairs, which permit de novo generation of three-dimensional models. The validity of our analysis is supported by the location of functionally important residues in highly constrained regions of the protein. Importantly, insect OR models exhibit a distinct transmembrane domain packing arrangement to that of canonical GPCRs, establishing the structural unrelatedness of these receptor families. The evolutionary couplings and models predict odour binding and ion conduction domains, and provide a template for rationale structure-activity dissection. In almost all of the many millions of insect species, repertoires of several dozen to several hundred highly divergent odorant receptors (ORs) are responsible for detecting a myriad of volatile chemical signals in the environment [1] . By transducing binding of specific odours into sensory neuron activity, insect ORs play critical roles in mediating olfactory behaviours such as mosquito host seeking [2] , moth mate identification [3] and drosophilid pathogen avoidance [4] . Surprisingly, the insect OR signalling mechanism has been challenging to define [5] , [6] . Like G protein-coupled receptors (GPCRs), insect ORs contain seven putative transmembrane helices (TMHs) [7] , [8] . This observation prompted a long-standing supposition that the insect receptors—similar to their mammalian counterparts—act metabotropically [8] , [9] , [10] , [11] , [12] . However, insect ORs have the opposite membrane orientation to GPCRs and function as heteromeric complexes (of unknown stoichiometry) of an odour ligand-specific ‘tuning’ OR and a co-receptor, ORCO (formerly called OR83b) [13] , [14] , [15] , [16] . Moreover, functional analyses in heterologous cells provided evidence that OR/ORCO complexes act as odour-gated cation channels [11] , [17] , [18] , [19] . However, the lack of similarity of insect ORs to known ion channel classes has made it difficult to dissect the molecular basis of this ionotropic function [20] . An important way to help resolve the mechanistic basis of insect OR signalling would be to obtain three-dimensional (3D) structural information of these receptors. Unfortunately, recombinant expression of these polytopic transmembrane proteins is technically very challenging [21] , which has precluded X-ray crystal structure determination. Furthermore, because insect ORs have no significant similarity to sequences of known 3D structure, homology modelling [22] , [23] is not possible. A complementary approach to predict both protein structure and functionally important sites is to use information contained within sequence variation among the members of large protein families [24] . Interactions between pairs of amino acids that are important for protein structure and function impose evolutionary constraints on the sets of mutations acceptable at interacting sites [25] . Reciprocally, identification of such evolutionary couplings (ECs) within primary sequences of isostructural proteins can provide information on distance restraints between amino acid pairs and thereby insight into higher-order structure and functional domains [25] . Identified coevolving residues can also, depending on the analysis method [25] , reflect distally coupled residues important for allosteric communication within proteins [26] , [27] . Here, we applied this approach to identify ECs across the large insect OR family, which we use to build de novo the first 3D models of these proteins and identify functionally important sites. We used an extended version of the EVfold-transmembrane method [28] ( Fig. 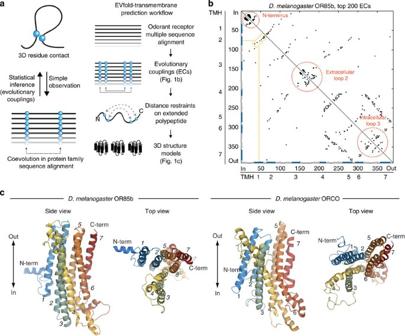Figure 1: Evolutionary couplings-derived insect OR models. (a) Left: the structural proximity of residues in a protein leaves a visible record of amino acid covariation in the protein family sequence alignment due to the evolutionary pressure to maintain favourable interactions. By analysing these patterns with a statistical model of sequence coevolution, ECs between residue pairs can be inferred and used to predict 3D contacts. Right: schematic of the EVfold-transmembrane prediction workflow (see Methods). A multiple alignment of insect OR protein sequences is used to identify ECs between pairs of coevolving amino acids with EVfold-PLM. After discarding pairs that are inconsistent with the predicted membrane topology and secondary structure, the remaining highest-ranking EC pairs are used as distance restraints on an extended polypeptide to fold a set of 3D OR models. (b) Contact map representation of the top 200 predicted ECs forD. melanogasterOR85b. The axes represent the indices along the OR85b primary sequence, along which predicted TMH segments are annotated as blue bars and predicted helical secondary structure as grey bars. Black dots represent ECs between pairs of residues; the representation is mirror-symmetric along the diagonal. The lines of ECs parallel and anti-parallel to the diagonal of the contact map are characteristic of the helix packing arrangements observed in alpha-helical transmembrane proteins28; the dashed orange lines highlights one of these between TMH1 and TMH2. Three high-density regions of ECs within the N-terminal tail, EL2 and IL3 are highlighted by red dashed circles (see alsoFig. 3a). (c) Top-ranked predicted 3D structural models for OR85b (left, model 140_12) and ORCO (right, model 310_2; the ORCO-specific IL2 insertion is not modelled) viewed from within the membrane bilayer (side view) and from the extracellular face (top view). Models are colour coded from N-terminus (blue) to C-terminus (red). As expected for members of the same protein family, the 3D models agree in their overall helical packing arrangement; the observed differences may be caused by actual structural differences of different subfamilies in the OR protein family sequence space and/or by inaccuracies in sequence alignment, statistical inference and 3D modelling. 1a ) to compute ECs for selected insect ORs, starting with multiple sequence alignments containing a set of 5,907 known and newly annotated receptors ( Supplementary Table 1 and Supplementary Data 1–4 ). From these alignments, we extracted patterns of amino acid coevolution to produce a ‘contact map’ of evolutionarily constrained pairs of residues along the OR sequence ( Fig. 1b , Supplementary Fig. 1 and Supplementary Data 5–8 ). These ECs were used in two ways: first, to probe functional sites, as evolutionary co-conservation reveals selection pressures beyond single position conservation ( Supplementary Data 9 and 10 ); second, to produce 3D models by combining ECs with secondary structure predictions to fold the OR polypeptide ( Fig. 1c and Supplementary Data 11–14 ). Figure 1: Evolutionary couplings-derived insect OR models. ( a ) Left: the structural proximity of residues in a protein leaves a visible record of amino acid covariation in the protein family sequence alignment due to the evolutionary pressure to maintain favourable interactions. By analysing these patterns with a statistical model of sequence coevolution, ECs between residue pairs can be inferred and used to predict 3D contacts. Right: schematic of the EVfold-transmembrane prediction workflow (see Methods). A multiple alignment of insect OR protein sequences is used to identify ECs between pairs of coevolving amino acids with EVfold-PLM. After discarding pairs that are inconsistent with the predicted membrane topology and secondary structure, the remaining highest-ranking EC pairs are used as distance restraints on an extended polypeptide to fold a set of 3D OR models. ( b ) Contact map representation of the top 200 predicted ECs for D. melanogaster OR85b. The axes represent the indices along the OR85b primary sequence, along which predicted TMH segments are annotated as blue bars and predicted helical secondary structure as grey bars. Black dots represent ECs between pairs of residues; the representation is mirror-symmetric along the diagonal. The lines of ECs parallel and anti-parallel to the diagonal of the contact map are characteristic of the helix packing arrangements observed in alpha-helical transmembrane proteins [28] ; the dashed orange lines highlights one of these between TMH1 and TMH2. Three high-density regions of ECs within the N-terminal tail, EL2 and IL3 are highlighted by red dashed circles (see also Fig. 3a ). ( c ) Top-ranked predicted 3D structural models for OR85b (left, model 140_12) and ORCO (right, model 310_2; the ORCO-specific IL2 insertion is not modelled) viewed from within the membrane bilayer (side view) and from the extracellular face (top view). Models are colour coded from N-terminus (blue) to C-terminus (red). As expected for members of the same protein family, the 3D models agree in their overall helical packing arrangement; the observed differences may be caused by actual structural differences of different subfamilies in the OR protein family sequence space and/or by inaccuracies in sequence alignment, statistical inference and 3D modelling. Full size image We used Drosophila melanogaster OR85b (a tuning OR that responds to 2-heptanone and several esters [29] , [30] ) and ORCO as anchors for these analyses to obtain models for both a ligand-specific OR and the co-receptor. ORs and ORCO have the same transmembrane topology [16] , [17] , [31] and can—with the exception of an ORCO-specific ~70 amino acid insertion in the intracellular loop 2 (IL2)—be confidently aligned over their whole length ( Supplementary Data 2 ). We therefore expect OR85b and ORCO to share the same overall 3D fold and our predicted ECs and structural models to be similar. However, differences in alignments arising from distinct anchor sequences that cover different parts of the sequence space of the protein family may capture subfamily-specific restraints [25] . Examination of the predicted contact maps for OR85b and ORCO revealed a number of lines of ECs parallel or perpendicular to the diagonal within predicted TMHs ( Fig. 1b , orange dashed box, and Supplementary Fig. 1 ), which are characteristic of parallel and anti-parallel helix arrangements in alpha-helical membrane proteins [28] . This observation provides one validation of our approach as the EC analysis is given no prior knowledge that insect ORs are transmembrane proteins. Importantly, the predicted helical contacts bear no resemblance to those of GPCRs or to those of the adiponectin receptor 1, a seven TMH protein that has the same membrane orientation as insect ORs [32] , but which appears to have a convergent helical arrangement to that of GPCRs ( Fig. 2 ) [28] . These observations indicate that insect ORs adopt a seven TMH packing arrangement that is distinct from GPCR structures. Thus, the shared heptahelical secondary structure of these receptor families is, in contrast to initial assumptions [8] , [9] , likely to be coincidental and not necessarily indicative of a shared signalling mechanism. 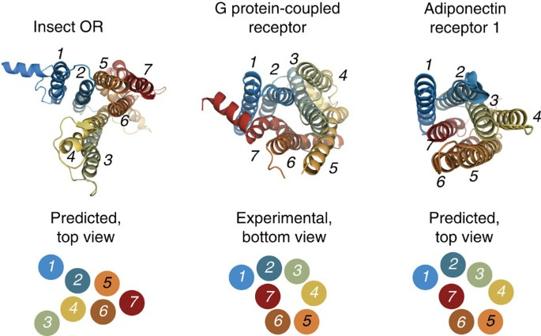Figure 2: An EC-based insect OR model has a heptahelical packing arrangement distinct from G protein-coupled receptors. Top:comparison of the helical packing arrangements of insect ORs, a GPCR and the adiponectin receptor 1 (AR1); the structures are colour coded from N-terminus (blue) to C-terminus (red). The OR is the top-ranked model of OR85b (seeFig. 1c); the GPCR is the crystal structure of the β2-adrenergic receptor (PDB 2RH1 (ref.55)); the AR1 structure is the top-ranked model described previously28. As the N-termini of ORs and AR1s are located in the cytosol, but the N-terminus of GPCRs is located extracellularly (or lumenally), the GPCR structure is shown in the opposite orientation so that the packing arrangements are visually comparable. Structures were rotated so that the positioning of TMH1 and TMH2 agrees, as far as possible, between the different molecules.Bottom:corresponding simplified two-dimensional representations of the helical contacts highlighting the difference between the helical packing arrangement of insect ORs when compared to GPCRs and AR1s. Figure 2: An EC-based insect OR model has a heptahelical packing arrangement distinct from G protein-coupled receptors. Top: comparison of the helical packing arrangements of insect ORs, a GPCR and the adiponectin receptor 1 (AR1); the structures are colour coded from N-terminus (blue) to C-terminus (red). The OR is the top-ranked model of OR85b (see Fig. 1c ); the GPCR is the crystal structure of the β2-adrenergic receptor (PDB 2RH1 (ref. 55 )); the AR1 structure is the top-ranked model described previously [28] . As the N-termini of ORs and AR1s are located in the cytosol, but the N-terminus of GPCRs is located extracellularly (or lumenally), the GPCR structure is shown in the opposite orientation so that the packing arrangements are visually comparable. Structures were rotated so that the positioning of TMH1 and TMH2 agrees, as far as possible, between the different molecules. Bottom: corresponding simplified two-dimensional representations of the helical contacts highlighting the difference between the helical packing arrangement of insect ORs when compared to GPCRs and AR1s. Full size image In analyses with both OR85b and ORCO, three regions of the sequences contain patches of residues with multiple, strong ECs (N-terminal tail, extracellular loop 2 (EL2) and intracellular loop 3 (IL3)/TMH7) ( Fig. 1b and Supplementary Fig. 1 , red dashed circles, and Fig. 3a ). These EC clusters suggest that these regions are under strong evolutionary constraint and are therefore predictive of functional importance [28] . Remarkably, although molecular insights into insect ORs are still in their infancy—and dispersed across several different ‘model’ receptors—experimental validation of the importance of all three regions is available. A single amino acid mutation in the N-terminus of the D. melanogaster pheromone receptor OR67d (C23W) abolishes receptor function in vivo [33] ; mapping of this residue onto the contact map by identifying the homologous position in OR85b (F11) and ORCO (A23) revealed it to lie within the N-terminal cluster of ECs ( Fig. 1b , Fig. 3a , Supplementary Fig. 1 and Supplementary Table 2 ), suggesting that this segment fulfils an important role in all ORs; we test this prediction below. The second patch of EC-enriched residues, in EL2, contains a number of predicted beta-turns separated by conserved proline residues; mutation of these, and adjacent residues, in several different ORs strongly or completely disrupts function [34] . Although our analysis is unable to predict the precise conformation of this loop, the presence of strongly constrained residues in this region is consistent with the detrimental effect of their mutation. Last, IL3 forms at least part of the molecular interface for assembly of ORCO and ligand-specific ORs into heteromeric complexes [16] , which may explain the very high frequency of strong ECs within this region ( Fig. 3a ). We are currently unable to distinguish ECs that mediate intramolecular versus inter-subunit interactions in these receptors. Nevertheless, a systematic mutational analysis of cysteine residues in D. melanogaster ORCO revealed a particularly important functional requirement for those cysteines in IL3 (ref. 35 ) ( Supplementary Table 2 ). In summary, although these observations do not validate the ECs and structural models per se , the striking coincidence of known functionally important sites with highly coupled residues gives basic confidence in our results. 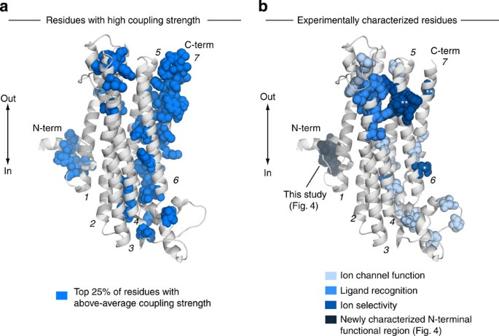Figure 3: Highly coupled OR residues coincide with experimentally characterized functional regions. (a) Positions with above-average EC strength (top 25% of sites, blue spheres) on the top-ranked model of OR85b (140_12;Supplementary Data 13; membrane-integral side view). Strongly coupled residues cluster around three regions of the model: (i) N-terminus, (ii) EL2, (iii) IL3 and along the span of TMH7. Many of the strongly coupled TMH7 residues do not feature in the contact map (Fig. 1b), because they were excluded as structural contacts with our standard transmembrane clash filter. (b) Experimentally characterized residues in different OR and ORCO proteins (spheres coloured by different shades of blue according to functional categorization;Supplementary Table 2) mapped onto the 3D model of OR85b (140_12), based on a sequence alignment of OR and ORCO sequences (Supplementary Data 2). Among many residues whose mutation have general deleterious effects on ion channel function, only a few residues influence ion selectivity (which are strong candidates for pore-lining residues), including two sites in ORCO (double asterisks marking residues at the extracellular end of TMH6 and TMH7) and two in a tuning OR (B. moriOR1) (single asterisks marking residues at the intracellular end of TMH5 and TMH6) (see text andSupplementary Table 2for details). Figure 3: Highly coupled OR residues coincide with experimentally characterized functional regions. ( a ) Positions with above-average EC strength (top 25% of sites, blue spheres) on the top-ranked model of OR85b (140_12; Supplementary Data 13 ; membrane-integral side view). Strongly coupled residues cluster around three regions of the model: (i) N-terminus, (ii) EL2, (iii) IL3 and along the span of TMH7. Many of the strongly coupled TMH7 residues do not feature in the contact map ( Fig. 1b ), because they were excluded as structural contacts with our standard transmembrane clash filter. ( b ) Experimentally characterized residues in different OR and ORCO proteins (spheres coloured by different shades of blue according to functional categorization; Supplementary Table 2 ) mapped onto the 3D model of OR85b (140_12), based on a sequence alignment of OR and ORCO sequences ( Supplementary Data 2 ). Among many residues whose mutation have general deleterious effects on ion channel function, only a few residues influence ion selectivity (which are strong candidates for pore-lining residues), including two sites in ORCO (double asterisks marking residues at the extracellular end of TMH6 and TMH7) and two in a tuning OR ( B. mori OR1) (single asterisks marking residues at the intracellular end of TMH5 and TMH6) (see text and Supplementary Table 2 for details). Full size image To validate the predictive power of our ECs in identifying important residues in insect ORs, we focussed on the N-terminal cytoplasmic region of ORCO, whose role (if any) is unknown. We generated a version of this receptor (ORCO 6Mut ) bearing mutations in six of the top-ranked constrained residues in the sequence of D. melanogaster ORCO (A23, M24, F30, M31, H32 and N33) ( Supplementary Data 10 ); several of these residues feature as pairs in the top-ranked ORCO ECs (that is, M24-F30, M24-M31 and M24-H32; Supplementary Data 6 ). We also generated an ORCO mutant bearing a small deletion spanning these residues (ORCO Δ23–33 ). Wild-type and mutant ORCO proteins were expressed in Xenopus oocytes for functional analysis by two-electrode voltage clamp recording of ligand-evoked current responses [20] . We first co-expressed ORCO with OR47a or OR85b, whose most potent agonists are pentyl acetate and 2-heptanone, respectively [18] , [30] , [36] . Wild-type ORCO co-expressed with these receptors can reconstitute dose-dependent odour-evoked currents ( Fig. 4a,b ). By contrast, ORCO 6Mut and ORCO Δ23–33 have highly diminished or abolished response to these odours, respectively ( Fig. 4a,b ). In a second set of experiments, we tested current responses of wild-type and mutant ORCOs to VUAA1, an artificial small-molecule agonist that can activate this co-receptor when expressed alone (without a tuning OR partner) [37] . Wild-type ORCO produced robust currents on VUAA1 presentation, but neither mutant protein responded to this ligand ( Fig. 4c ). Taken together, our computational and experimental data support a previously unappreciated function for the ORCO N-terminus; that the tuning receptor OR67d is also sensitive to a mutation in this region [33] suggests that this sequence may have a conserved role across the OR family. Determining the precise contribution of the N-terminus to receptor function—for example, in folding, trafficking and/or complex assembly—will nevertheless require further experimentation beyond the scope of this study. 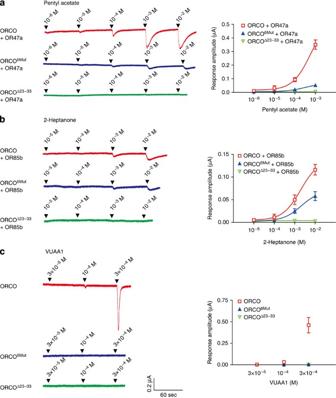Figure 4: Functional analysis of the ORCO N-terminus. (a–c) Left: representative whole-cell current traces to the indicated stimuli with two-electrode voltage-clamp inXenopusoocytes injected with cRNAs for the indicated combinations of wild-type or mutantD. melanogasterORs. ORCO6Mutcontains amino acid substitutions in the six top-ranked N-terminal residues (A23S, M24A, F30A, M31A, H32A and N33A); ORCOΔ23–33bears a deletion of this region (A23–N33). Ligand solutions were applied for 3 s (arrowheads). Right: quantification of current amplitudes (mean±s.e.m.;n=5 oocytes for wild-type ORCO and ORCO6Mut;n=4 for ORCOΔ23–33). Figure 4: Functional analysis of the ORCO N-terminus. ( a – c ) Left: representative whole-cell current traces to the indicated stimuli with two-electrode voltage-clamp in Xenopus oocytes injected with cRNAs for the indicated combinations of wild-type or mutant D. melanogaster ORs. ORCO 6Mut contains amino acid substitutions in the six top-ranked N-terminal residues (A23S, M24A, F30A, M31A, H32A and N33A); ORCO Δ23–33 bears a deletion of this region (A23–N33). Ligand solutions were applied for 3 s (arrowheads). Right: quantification of current amplitudes (mean±s.e.m. ; n =5 oocytes for wild-type ORCO and ORCO 6Mut ; n =4 for ORCO Δ23–33 ). Full size image Finally, we asked whether our analysis could provide insight into the proposed function of insect ORs as ligand-gated ion channels. Four studies have experimentally defined mutations that affect (directly or indirectly) ligand recognition properties of different receptors [30] , [38] , [39] , [40] ( Supplementary Table 2 ). Notably, when mapped onto the OR85b model, these cluster in the external half of the TM2-4 region ( Fig. 3b ), suggesting that this region comprises a part of a ligand-binding pocket. The proposition that the relatively long EL2 loop might form a ‘lid’ that could cover/uncover this pocket [34] is inline with the location of these residues. Although ORs do not bear strong similarity to known ion channels, previous characterization of a sequence suggested to bear some resemblance to a K + channel selectivity filter in D. melanogaster ORCO TMH6 (T 393 VVGYLG 399 ) demonstrated a role in controlling K + permeability [11] ( Supplementary Table 2 ). Independently, a systematic screen of residues in Bombyx mori ORCO showed mutation of Y464 (in TMH7)—and the equivalent Y478 in D. melanogaster ORCO—affected K + selectivity [20] . Strikingly, this residue lies directly opposite the TVVGYLG sequence in our model, suggesting that this region forms a key part of the pore ( Fig. 3b , double asterisks). Channel properties depend on both ORCO and the tuning OR, indicating that both subunits contribute to formation of the ion-conducting passage [18] , [20] , [41] , [42] . We therefore mapped the position of additional residues that have direct or indirect effects on channel function [20] ( Supplementary Table 2 ). The majority of these are in TMH5-7 region ( Fig. 3b ), consistent with this region forming a central part of the ion-conducting channel; notably, the only two of these residues that have effects on K + ion selectivity (D299 and E356 in B. mori OR1; ref. 20 )—as opposed to more general deleterious effects on ion channel function—are also located directly opposite to each other at the cystosolic end of TMH5 and TMH6 ( Fig. 3b , single asterisks). Future determination of the stoichiometry of the heteromeric complex and identification of inter-subunit ECs may permit modelling of its quaternary structure to visualize how this C-terminal region forms the ion-conducting channel. The function of these receptors in odour-evoked signalling clearly depends on other regions too, such as the N-terminus and EL2. Our analysis of ECs in insect ORs has allowed us to build the first 3D models of this receptor family. These proteins appear to define a novel fold, as searches with DALI [43] did not reveal highly significant similarity of our models to experimentally determined membrane protein structures (data not shown). It is, however, important to keep in mind that our current models are coarse grained, and the accuracy of the folded 3D structures is limited by multiple factors, including: (i) the availability of OR sequences, (ii) accurate secondary structure predictions and (iii) the confounding of monomer folding by the presence of multimer contacts, conformational plasticity and functional couplings, which are not easily disambiguated. As additional receptor sequences become available and as the EVfold method itself is further developed to fold multimers, future OR models—which we plan to update on the EVfold website ( http://evfold.org )—will be more accurate. It will be of particular interest to determine whether ORCO and ligand-specific ORs have distinct structural features. For ORCO-specific predictions, many hundreds of additional ORCO sequences from other insects are required. Similarly, increased sequence availability and improvement of alignments will aid analysis of the divergent tuning ORs. Nevertheless, the current models are both consistent with available and new experimental data and offer a number of predictions—notably, through revelation of highly constrained residues ( Supplementary Data 9 and 10 )—to guide and visualize structure–function analyses of these unusual sensory receptors. Moreover, these predictions may be the first step to assist in the design of novel pharmacological reagents to manipulate OR function, and thereby control olfactory behaviours of pest insects. Annotation of OR sequences New OR sequences from nine additional drosophilid genomes ( Supplementary Table 1 and Supplementary Data 1 ) were identified by TBLASTN [44] using D. melanogaster OR protein sequences as queries. Multiple sequence alignment All identified OR sequences were compiled into a FASTA database ( Supplementary Data 1 ) and aligned iteratively with either D. melanogaster OR85b or D. melanogaster ORCO as reference sequences using jackhmmer with default parameters [45] . In the ORCO-anchored alignment, homologues that split into two separate aligned domains (due to the presence of the ORCO-specific insertion in IL2) were re-merged using custom Python scripts. In the OR85b-anchored alignment, the inclusion E-value (1E-40) was manually chosen to maximize EC contrast over residual background couplings. In both cases, alignment columns with >50% gaps were excluded from EC analysis as described [28] . ECs inference from sequence variation ECs were calculated with an updated version of our protocol (EVfold-PLM) based on a pseudolikelihood maximization statistical inference procedure [46] , [47] , [48] instead of the original mean-field approximation [24] . Sequences in the alignment were downweighted at a 90% identity threshold to reduce the influence of sampling bias on statistical inference. Webserver and code for EC calculations are available on evfold.org. De novo folding from protein sequences The folding protocol is described in more detail elsewhere [24] , [28] . In brief, ECs were filtered using a combination of predicted transmembrane topology and predicted secondary structure. Transmembrane topology was predicted using PolyPhobius [49] and validated by consensus prediction using TOPCONS [50] and MEMSAT-SVM [51] . Secondary structure was predicted using PSIPRED [52] and low confidence predictions of helix or beta-strand in ORCO (reliability index <3) were set to coil. Increasing numbers of top-ranked ECs were then used to fold D. melanogaster OR85b and ORCO from an extended polypeptide with CNS distance geometry and simulated annealing [53] . Local secondary structure was constrained based on the predicted topology and secondary structure. Due to the lack of alignment coverage on the ORCO-specific insertion in IL2 (residues 247–329), this region was not modelled to avoid interference with the folding of the membrane integral domain. Clustering and ranking of predicted models All generated protein models were clustered and ranked using the default quality assessment protocol of EVfold-transmembrane [24] , [28] . The ranking procedure uses a score composed of the agreement of each model with predicted lipid exposure, predicted secondary structure, and ECs. Models with structural knots are excluded from consideration as top-ranked models. Additional structure-based clustering ensures that high-scoring outlier structures can be excluded from consideration as confident predictions. Model visualization and annotation Protein models were visualized and annotated using PyMOL Molecular Graphics System, Version 1.5.0.4 Schrödinger, LLC. To annotate functionally analysed residues of different ORs ( Supplementary Table 2 ) on the common model, the equivalent positions in OR85b and ORCO were determined using the jackhmmer multiple sequence alignment anchored around OR85b ( Supplementary Data 2 ). Functional analysis of ORs in Xenopus oocytes Mutant orco plasmid constructs were generated by standard cloning procedures; primer sequences are as follows: ORCO 6Mut (forward: 5′-GCGCGAATTCGCCACCACCATGACAACCTCGATG-3′, reverse: 5′-CAGGCCGGAGTACTTCGCCGACCGGATGTTGGGCAT-3′; and forward: 5′-AAGTACTCCGGCCTGGCCGCGGCCGCCTTCACGGGCGGCAGT-3′, reverse: 5′-GCGCCTCGAGTTACTTGAGCTGCAC-3′) and ORCO Δ23–33 (forward: 5′-TTCACGGGCGGCAGTGCCTTC-3′, reverse: 5′-CCGGATGTTGGGCATCAGGTC-3′). cRNAs were synthesized from linearized modified pSPUTK vector [54] containing wild-type or mutant versions of D. melanogaster ORCO, OR47a or OR85b. Stage V–VII oocytes were treated with 2 mg ml −1 of collagenase B (Roche Diagnostics, Tokyo, Japan) in Ca 2+ -free saline solution (82.5 mM NaCl, 2 mM KCl, 1 mM MgCl 2 and 5 mM HEPES, pH 7.5) for 1–2 h at 18 °C. Oocytes were microinjected either with 6.25 ng cRNA encoding a ligand tuning OR (OR47a or OR85b) and 6.25 ng cRNA encoding ORCO ( Fig. 4a,b ) or 12.5 ng of ORCO cRNA ( Fig. 4c ). Injected oocytes were incubated for 3–4 days at 18 °C in Barth’s solution supplemented with 84.7 mg l −1 of gentamycin. Whole-cell currents were recorded using the two-electrode voltage-clamp technique as previously described [3] . Intracellular glass electrodes were filled with 3 M KCl. Signals were amplified with an OC-725C amplifier (Warner Instruments, Hamden, CT, USA), low-pass filtered at 50 Hz and digitized at 1 kHz. Ligand solution was delivered via a silicon tube connected to a computer-driven solenoid. Before experiments, pentyl acetate (CAS: 628-63-7; Wako, Osaka, Japan) and 2-heptanone (CAS: 110-43-0; TCI, Tokyo, Japan) were directly diluted into the bath solution (115 mM NaCl, 2.5 mM KCl, 1.8 mM BaCl 2 and 10 mM HEPES, pH 7.2). VUAA1 (CAS: 525582-84-7; Vitas-M Laboratory, Moscow, Russian Federation) was prepared in dimethylsulphoxide as 20 mM, 66.7 mM or 200 mM stock solutions, which were then diluted into the bath solution at 0.15% to give the final desired concentration. How to cite this article : Hopf, T. A. et al. Amino acid coevolution reveals three-dimensional structure and functional domains of insect odorant receptors. Nat. Commun. 6:6077 doi: 10.1038/ncomms7077 (2015).